High-pressure synthesis of a polyethylene/zeolite nano-composite material Meso/micro-porous solids, such as zeolites, are complex materials used in an impressive range of applications. Here we photo-polymerized ethylene using non-catalytic high-pressure techniques at 0.5–1.5 GPa under ultraviolet (351–364 nm) irradiation on a sub-nanometre scale in the channels of a pure SiO 2 zeolite, silicalite, to obtain a unique nano-composite material with drastically modified mechanical properties. The structure obtained contains single polyethylene chains, which adapt very well to the confining channels as shown by optical spectroscopy and X-ray diffraction. The formation of this nano-composite results in significant increases in bulk modulus and density, and the thermal expansion coefficient changes sign from negative to positive with respect to silicalite. Mechanical properties may thus be tuned by varying the amount of polymerized ethylene. Our findings could allow the high-pressure, catalyst-free synthesis of a unique generation of technological, functional materials based on simple hydrocarbons polymerized in confining meso/micro-porous solids. Meso/micro-porous materials can be considered as very small chemical laboratories, where chemical reactions are induced and controlled on a small scale down to just a few angstroms. Their large-scale applications are, among others, fine gas separation, gas storage and catalysis [1] , [2] , [3] , [4] , [5] , [6] , [7] , [8] , [9] . More emerging applications of these materials, once properly functionalized, are also in sight in diverse fields such as nano-electronics, nano-sensoring and nano-photonics [10] , [11] . A very intriguing aspect of ordered nano- and subnano-porous solids is the ability to drive the formation of confined polymers with remarkable physical properties (see [12] , [13] , [14] , [15] , [16] , [17] and other references therein). Polymerization is usually performed by complex chemical methods including the use of catalysts and radical initiators, which are either supplied by the wall of the nano-pores or are added to the pores together with the reactants. This type of chemistry was used, for instance, to encapsulate conducting filaments of polyaniline [18] and graphite-type carbon wires [19] in the 3-nm-wide ordered hexagonal channel system of the porous aluminosilicate MCM-41. Crystalline linear polyethylene (PE) nano-fibers have also been produced by catalysed polymerization and extrusion through meso-porous silica [20] . The goal of this study is to push the effect of confinement on polymerizing matter down to the sub-nanometre scale, while avoiding any catalytic effects from the pore walls to better understand the effect of confinement per se and to fully characterize these materials from a structural point of view. Unique nano-composite materials could be synthesized in this way. A strong advantage of high-pressure polymerization techniques with respect to more conventional catalytic protocols is precisely that these techniques allow the use of catalysts and radical initiators to be avoided [21] , [22] , [23] , which is indispensable to determine the intrinsic role of spatial confinement on polymerizing matter. Indeed, pressure is the most efficient tool to reduce intermolecular distances, thereby permitting continuous tuning of the corresponding interactions and allowing the chemical reactions to occur, which are in some cases enhanced by ultraviolet (UV) light irradiation, when a critical intermolecular distance is approached in this way [24] . Another strong advantage of the high-pressure methodology in synthesizing composite materials is that once these procedures are scaled up to provide sufficiently large amounts of product material, they could represent a true, novel ‘green chemistry’ route to industrial chemical synthesis, as the use of additional and polluting compounds such as the catalysts and radical initiators is avoided. The best candidate as the host material for our purpose to synthesize a nano-composite material can be found among zeolites. These materials are micro-porous, crystalline, inorganic solids made of corner-sharing SiO 4 and AlO 4 tetrahedra with strong acid character and catalytic properties. At one end of this class, there is silicalite, which is an electrically neutral, non-catalytic pure SiO 2 zeolite. Silicalite is characterized by a framework of 4-, 5-, 6- and 10-membered rings of corner-sharing SiO 4 tetrahedra forming interconnected, mutually orthogonal straight and sinusoidal 5.5 Å diameter channels (see [25] and references therein). Silicalite can easily adsorb simple molecules, such as Ar, CO 2 [26] , [27] , [28] ), and straight n-alkanes (up to n =10), and, interestingly, computer simulations indicate that n-alkane chains easily adapt to the channels [29] , [30] . We then chose ethylene as a benchmark, simple hydrocarbon to undergo polymerization in the sub-nano channels of silicalite with the aim of producing a unique nano-composite material. To our knowledge, ethylene was never polymerized in a nano-confining host material, neither by catalytic nor by non-catalytic routes. Polymerization was induced by applying pressures of 0.5–1.5 GPa to the confined reactant and using UV irradiation (351–364 nm) as an optical catalyst, which we have already shown to be efficient conditions for polymerizing bulk ethylene and other simple hydrocarbons [21] , [22] , [23] . The composite was characterized by optical spectroscopy, and single-crystal and powder X-ray diffraction (XRD). The structure obtained contains single PE chains, which adapt very well to the confining channels and strongly modify the mechanical properties of the host zeolite. Here and in the following the nano-composite product material will be referred to as PESIL, from PE and SIL (silicalite). Synthesis of PESIL Supercritical fluid ethylene was loaded in a diamond anvil cell (DAC) and compressed to 0.5–1.5 GPa, at room temperature, together with either polycrystalline or single-crystal silicalite-1F. A total of four samples were prepared in this way. In the polycrystalline case, finely ground silicalite powder almost completely filled the sample thickness (40–80 μm), so that the vast majority of the loaded ethylene occupied the micropores, and only a small remaining amount was found in the interstitial spaces as bulk C 2 H 4 . In the second case, a single crystal of typically 40 × 40 × 80 μm 3 was placed in the gasket that was then filled with ethylene, which entered into the pores and also formed a bulk, surrounding domain. Ethylene completely filled the pores of silicalite, as has previously been found for other small molecules and atoms such as Ar and CO 2 (refs 26 , 27 , 28 ). In fact, gas adsorption in silicalite reaches saturation at typical pressures well below the liquid–vapor transition pressure [30] , whereas our compressed fluid is about 25% denser than the liquid phase. The Raman active C=C stretching mode of ethylene at about 1,628 cm −1 shows a clear signature of the micro-confined molecules ( Fig. 1 ). The bands of bulk and confined ethylene are split by about 8% and that of the confined molecules is much broader. This indicates the presence of a moderate interaction between C 2 H 4 and the silicalite wall surface, which did not lead to significant chemical reactivity. The polymerization of ethylene was then performed at 0.5–1.5 GPa under UV irradiation (CW Ar + laser, at 351–364 nm) for a few hours with typical power density of 1.6–3.2 W mm −2 . Polymerization and the obtained PESIL were investigated by Raman and IR absorption spectroscopy, and powder and single-crystal XRD. 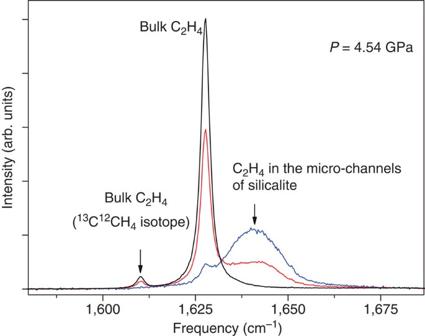Figure 1: Raman spectra of the C=C stretching line of ethylene. Measurement was performed at 4.54 GPa on a mixture of C2H4and silicalite-1F single crystals. (i) Black spectrum, measured on bulk ethylene (thickness of about 40 μm); (ii) red spectrum, measured on a silicalite crystal with bulk ethylene on the top (C2H4thickness of about 10 μm); (iii) blue spectrum, measured on the top of a silicalite crystal, which is nearly bridging the two diamond anvils (C2H4thickness of less than 1 μm). Sharp peaks at about 1,628 cm−1and 1,610 cm−1:12C=12C and13C=12C stretching lines of bulk C2H4, respectively. Broad peak at about 1,641 cm−1:12C=12C stretching band of ethylene confined in the micro-channels of silicalite. The three spectra have been normalized to the same integrated intensity. Ethylene is in solid phase I and we did not observe spontaneous chemical reactions at the typical time scale (1–2 h) of the Raman investigation (see also in31). Figure 1: Raman spectra of the C=C stretching line of ethylene. Measurement was performed at 4.54 GPa on a mixture of C 2 H 4 and silicalite-1F single crystals. (i) Black spectrum, measured on bulk ethylene (thickness of about 40 μm); (ii) red spectrum, measured on a silicalite crystal with bulk ethylene on the top (C 2 H 4 thickness of about 10 μm); (iii) blue spectrum, measured on the top of a silicalite crystal, which is nearly bridging the two diamond anvils (C 2 H 4 thickness of less than 1 μm). Sharp peaks at about 1,628 cm −1 and 1,610 cm −1 : 12 C= 12 C and 13 C= 12 C stretching lines of bulk C 2 H 4 , respectively. Broad peak at about 1,641 cm −1 : 12 C= 12 C stretching band of ethylene confined in the micro-channels of silicalite. The three spectra have been normalized to the same integrated intensity. Ethylene is in solid phase I and we did not observe spontaneous chemical reactions at the typical time scale (1–2 h) of the Raman investigation (see also in [31] ). Full size image Characterization of PESIL by IR spectroscopy IR spectroscopy shows that ethylene undergoes polymerization giving rise to almost 100% conversion of the reactant over a few hours ( Fig. 2a ). The sample was then recovered at ambient pressure and further investigated ( Fig. 2b ). The IR spectrum provides important information on the structure of the confined PE as seen, for instance, in the spectral region of the intense CH 2 bending mode doublet at 1,463–1,473 cm −1 . The structure of the doublet is characteristic of an ordered orthorhombic crystal ( Pnam , Z =2). In the case of high-pressure, UV-assisted polymerization of bulk ethylene, this doublet is by far the dominant feature between 1,300 and 1,500 cm −1 (ref. 21 ). In our case, when either part or almost the full sample region is occupied by silicalite powder, we observe in the middle of the sharp doublet, due to bulk PE, a strong and broad single-chain bending peak at 1,468 cm −1 with shoulders at 1,458 and 1,445 cm −1 , and two broad wagging mode bands at 1,353 and 1,370 cm −1 . The shoulders and the wagging peaks, which are very weak in the bulk polymer [21] , [31] , are entirely due to gauche defects. All these peaks correspond to disordered PE with gauche defects among others, which we assign to confined PE in the micro-channels of silicalite. It is thus evident that some strain is imposed on the polymeric chains due to the high degree of confinement. In addition, the relatively sharp, weak peak at 1,379 cm −1 is due to the methyl groups of confined PE. This implies the presence of a few relatively short branched chains, which are probably related to crystalline defects in silicalite. 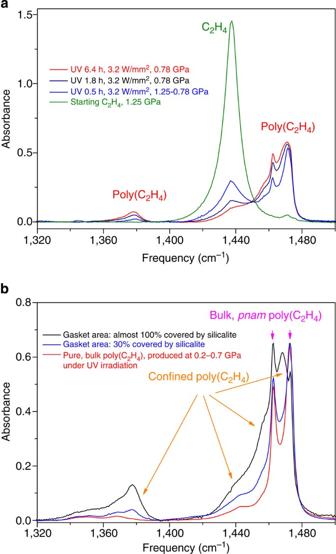Figure 2: IR absorption spectra in a selected frequency region showing the formation of confined and bulk polyethylene. (a) The sample region is almost fully occupied by silicalite powder. Pressures: 0.78–1.25 GPa. Olive: starting sample showing the strong CH2bending peak of ethylene at 1,437 cm−1and a very small amount of the corresponding polyethylene peak at 1,470 cm−1due to a very small, accidental initial laser irradiation. Blue, navy and red: the same sample after 0.5, 1.8 and 6.4 h of UV irradiation, respectively, showing the progressive formation of polyethylene at the expense of ethylene. (b) Final (recovered and ambient pressure) mixtures of polyethylene and silicalite powder with the silicalite occupying almost the full sample thickness and about 30% (blue) and 100% (black) of the sample area exposed to the incoming IR beam. Red: a pure polyethylene sample obtained under pressure and UV irradiation21. The sharp doublet at 1,463–1,473 cm−1is due to bulk polyethylene, while all the other peaks are mainly due to highly strained, confined polyethylene chains in the micro-channels of silicalite. The three spectra are normalized to the same peak absorbance at 1,450–1,480 cm−1. Figure 2: IR absorption spectra in a selected frequency region showing the formation of confined and bulk polyethylene. ( a ) The sample region is almost fully occupied by silicalite powder. Pressures: 0.78–1.25 GPa. Olive: starting sample showing the strong CH 2 bending peak of ethylene at 1,437 cm −1 and a very small amount of the corresponding polyethylene peak at 1,470 cm −1 due to a very small, accidental initial laser irradiation. Blue, navy and red: the same sample after 0.5, 1.8 and 6.4 h of UV irradiation, respectively, showing the progressive formation of polyethylene at the expense of ethylene. ( b ) Final (recovered and ambient pressure) mixtures of polyethylene and silicalite powder with the silicalite occupying almost the full sample thickness and about 30% (blue) and 100% (black) of the sample area exposed to the incoming IR beam. Red: a pure polyethylene sample obtained under pressure and UV irradiation [21] . The sharp doublet at 1,463–1,473 cm −1 is due to bulk polyethylene, while all the other peaks are mainly due to highly strained, confined polyethylene chains in the micro-channels of silicalite. The three spectra are normalized to the same peak absorbance at 1,450–1,480 cm −1 . Full size image Characterization of PESIL by XRD While optical spectroscopies give important information on the structure of PESIL, XRD using single-crystal data obtained from a typical sample recovered at ambient pressure is the most suitable technique to determine its crystal structure ( Table 1 and Supplementary Tables S1 and S2 ). Starting from the Pnma structural model for the SiO 2 framework, the C atoms were located from Fourier difference maps giving a total of 68 C atoms per unit cell. This indicates that before polymerization silicalite contained 34 molecules of ethylene per unit cell, which is significantly higher than the 11 molecules per unit cell typically obtained by gas adsorption [32] . The resulting structure is unique ( Fig. 3 and Supplementary Fig. S1 ) in terms of the arrangement of single PE chains within the confining channels. Four single, ideally infinite PE chains form inside the unit cell of silicalite, each having 17 C atoms per unit cell, and adapt fairly well to the shape of the 10-membered ring channels, whereas the smaller channels do not contain PE, because of steric hindrance. However, these chains are affected by a high degree of strain as a result of the nano-confinement. Two straight, zig–zag chains lie in the straight channels along b with the carbon atoms remarkably displaced from the plane containing what should be the ideal zig–zag skeletal C chain [33] . The other two chains lie in the two sinusoidal channels in the ac plane. In this case, not only do the carbon atoms deviate from the skeletal plane, but the chains are also sinusoidal to follow the sinusoidal shape of the confining channels. Importantly, there are no interconnections between the two types of polymeric chains. Confined PE is not commensurate with the host channels, because of the strong strain-related disorder. The large atomic displacement parameters ( Supplementary Table S2 ) can be expected to correspond to static distributions of the occupation of the carbon atoms in the pore and thus to translational and some rotational static disorder of the PE chains. The presence of defects in confined PE, as indicated by IR spectroscopy, is thereby confirmed by the structural analysis. Another spectacular aspect of PESIL is the remarkable change found in the structure of the SIL host with respect to that of pure, ambient pressure monoclinic silicalite. As in the case of silicalite filled by Ar and CO 2 under pressure [26] , the unit cell metric is now almost pseudo-tetragonal with the a and b lattice parameters only differing by 0.1% and the PE-filled silicalite cell volume is about 2% larger than that of the empty pure SiO 2 cell. The volume thermal expansion coefficient was found to be 7 × 10 −5 K −1 based on variable temperature XRD measurements. This is also surprising as filling with PE has the effect of changing the sign of the thermal expansion coefficient of orthorhombic SIL from a negative [8] , [9] to a normal positive value, which is close to twice that of quartz and one order of magnitude lower than that of ultra high molecular-weight pure PE (UHMWPE). Table 1 Single-crystal data and bulk modulus of PESIL ((SiO 2 ) 96 (C 2 H 4 ) 34 , space group Pnma ). 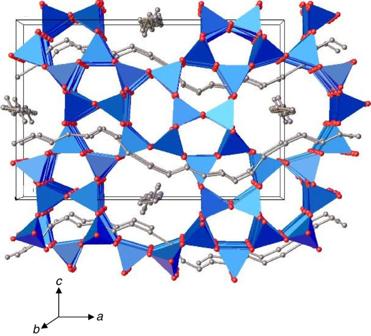Figure 3: Structure of PESIL (space groupPnma) obtained by single-crystal XRD. Blue polyhedra: SiO4tetrahedra; red spheres: O atoms; grey spheres: C atoms. Hydrogen atoms are not shown. Four ideally infinite polyethylene chains form in the unit cell of silicalite: two straight ones along thebaxis and two sinusoidal ones in theacplane. There are no interconnections between the two types of polymeric chains. The polymer chains are severely strained and not commensurate with silicalite. See alsoSupplementary Figure S1. Full size table Figure 3: Structure of PESIL (space group Pnma ) obtained by single-crystal XRD. Blue polyhedra: SiO 4 tetrahedra; red spheres: O atoms; grey spheres: C atoms. Hydrogen atoms are not shown. Four ideally infinite polyethylene chains form in the unit cell of silicalite: two straight ones along the b axis and two sinusoidal ones in the ac plane. There are no interconnections between the two types of polymeric chains. The polymer chains are severely strained and not commensurate with silicalite. See also Supplementary Figure S1 . Full size image The mechanical properties of PESIL were determined by measuring the XRD patterns as a function of pressure at room temperature on the polycrystalline sample. The equation of state (EOS) was obtained along with a test of resistance against pressure-induced amorphization [25] ( Fig. 4 ). The XRD pattern of silicalite strongly changes when it is filled by ethylene under pressure, as observed before inducing polymerization ( Fig. 4a ): the low angle peaks below 5° remarkably weaken with respect to those above 8° as a result of changes in structure factor due to the presence of C 2 H 4 . This trend was already observed in the case of silicalite filled with CO 2 and Ar at high pressures and is another proof that the host micro-channels are filled with guest molecules [26] , [27] . After polymerization, PESIL was investigated under pressure up to 24 GPa. The XRD pattern still exhibits Bragg peaks at the maximum pressure, thereby showing that pressure-induced amorphization of the host silicalite, which occurs progressively in pure silicalite and is complete at about 8 GPa, is prevented by the encapsulated PE, which is similar to what was also observed with CO 2 and Ar as guest species [26] . An accurate EOS is obtained upon compression up to 6 GPa ( Fig. 4b and Table 1 ), above which PESIL is affected by strong metastabilities, which are probably due to the non-hydrostatic compression. Silicalite-1-F is highly compressible, with a bulk modulus ( B 0 ) of 13.6 GPa [25] . Pressure–volume data for PESIL can be fitted to a third order Birch–Murnagam EOS [34] with a B 0 value of 26.7(2.0) GPa and the first derivative ( B 0 ’) of 4 ( Table 1 ). The encapsulated PE in PESIL thus remarkably increases the bulk modulus to a value, which is closer to that of α-quartz [35] , as in the case of CO 2 - and Ar-filled silicalite [26] . In addition, the density of PESIL is 2.054 (1) g cm −3 , which is lower than that of α-quartz by about 22%, mainly because it is a SiO 2 /C n H 2n composite material. 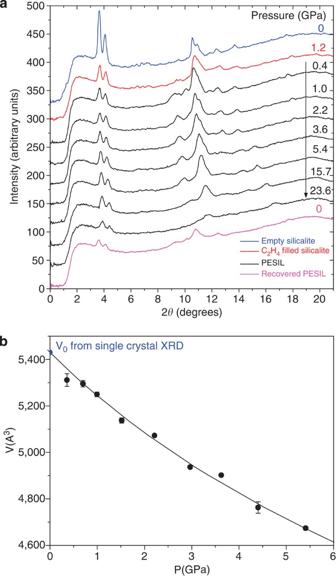Figure 4: Powder XRD on PESIL upon pressure increase. (a) XRD patterns of empty silicalite-1F (blue), ethylene-filled silicalite before polymerization (red), PESIL under pressure (black) and PESIL recovered at ambient pressure after compression (magenta); (b) equation of state: unit cell volume data versus pressure. Figure 4: Powder XRD on PESIL upon pressure increase. ( a ) XRD patterns of empty silicalite-1F (blue), ethylene-filled silicalite before polymerization (red), PESIL under pressure (black) and PESIL recovered at ambient pressure after compression (magenta); ( b ) equation of state: unit cell volume data versus pressure. Full size image High-pressure techniques permitted PESIL to be synthesized without catalysts producing a unique nano-composite material made of a pure SiO 2 zeolite filled by single PE chains. The new material was recovered at ambient pressure. PESIL is crystalline, although the polymeric chains are strained and disordered as a result of nano-confinement. In fact, the polymers are strained in such a way to adapt fairly well to the confining channels of silicalite. PESIL exhibits interesting mechanical properties: (i) it is only 28% softer than α-quartz, but stiffer than silicalite and UHMWPE by about a factor of 2 and 5, respectively; (ii) it exhibits a volume thermal expansion coefficient close to twice that of α-quartz, but which is lower than that of UHMWPE by one order of magnitude; and (iii) it is 22% less dense than α-quartz, whereas it is 15% denser than silicalite and about a factor of 2.2 denser than UHMWPE. It is particularly interesting that the polymerization of ethylene in silicalite changes the sign of the thermal expansion coefficient from negative to positive. The index of refraction of PESIL could also exhibit intermediate values between those of silicalite and quartz. In principle, PESIL or similar composite materials can be produced with a variety of well-tailored mechanical properties, which could be tuned either by changing the amount of ethylene polymerized in the micro-channels of silicalite or by changing the host zeolite. Particularly, a zero thermal expansion version of PESIL could be synthesized. These findings, together with the moderately high pressures needed for the synthesis of PESIL, could open the way for the large-scale production of a new variety of composite materials with interesting technological applications as supports for optics in aerospace devices among others. Even more sophisticated applications could be in sight. The potential high-pressure, catalyst-free synthesis of nano-composite materials similar to PESIL, but based on conducting polymers along with the potential high-pressure functionalization of zeolite micro-channels could open the way to an entirely new class of micro/nano-structured materials uniquely suited for advanced electronic and photonic applications. For instance, high-pressure polymerization could lead to the incorporation of conducting polymers, such as polyacetylene, which would be well protected in the zeolite matrices and are not chemically stable otherwise. This would in turn result in the production of novel, ideal conducting organic/inorganic composite materials. Optical spectroscopy methods IR spectra were measured using a Bruker IFS-120 HR Fourier transform infrared spectrometer equipped with an optical beam condenser based on ellipsoidal mirrors [36] . Raman spectra were performed using the 647.1-nm line of a Kr + laser as the excitation source. Backscattering geometry was used with X20 Mitutoyo micro-objective, and the signal was detected by an Acton/SpectraPro 2500i single monochromator, equipped with a CCD detector (Princeton Instruments Spec-10:100 BR). Powder XRD methods Angle dispersive, powder XRD patterns were obtained using a Mo micro-source ( λ =0.71073 Å), equipped with multilayered focusing mirrors (Xenocs-GeniX Mo Small Spot). The final X-ray spots on the sample and beam divergence were 100 μm and 0.2°, respectively. The diffracted signal was detected by a CCD detector (PI-SCX 4300). Typical integration time for each pattern was 1 h. The diffraction patterns were then analysed and integrated using the FIT2D program [37] . Single-crystal XRD methods Single-crystal XRD measurements were performed using Cu K α radiation ( λ =1.54185 Å) with an Agilent Gemini Diffractometer equipped with a Sapphire CCD detector at 70.00 mm. The single crystal was studied directly in the stainless steel gasket after the high-pressure synthesis. Low temperatures were obtained by cooling the sample in a cold nitrogen jet using an Oxford Instruments Cryojet device. Data collection, indexing and reduction were performed using CrysalisPro (Agilent Technologies). Absorption corrections for the crystal and the bulk PE and gasket shadowing corrections implemented in the software package Absorb 6.0 (ref. 38 ) were performed. Structure refinements were performed using SHELXL97 (ref. 39 ). Twinning defined by a twofold twin axis along the [110] direction was taken into account. Due to the high degree of disorder in the PE chains, constraints were added for the C-C distances and the isotropic atomic displacement parameters (ADPs) of the different sets of C atoms on general positions were constrained to be equal. High-pressure methods DACs were used for the high-pressure experiments, with typical sample diameter and thickness of 250 and 30–80 μm, respectively. Ethylene (purity 99% from Rivoira) was loaded in the DAC cryogenically in the liquid phase at −20 °C and 30 bar together with powdered or single crystal, hydrophobic hydrogen-free silicalite-1-F (SOMEZ, France). A ruby chip was put in the sample chamber for pressure measurements, using the ruby fluorescence method [40] . Accession codes: the X-ray crystallographic coordinates for structures reported in this article have been deposited at the Cambridge Crystallographic Data Centre (CCDC), under deposition number CCDC 919628. These data can be obtained free of charge from The Cambridge Crystallographic Data Centre via www.ccdc.cam.ac.uk/data_request/cif . How to cite this article: Santoro, M. et al . High-pressure synthesis of a polyethylene/zeolite nano-composite material. Nat. Commun. 4:1557 doi: 10.1038/ncomms2564 (2013).